iPSC-derived neurons from GBA1-associated Parkinson’s disease patients show autophagic defects and impaired calcium homeostasis Mutations in the acid β-glucocerebrosidase ( GBA1 ) gene, responsible for the lysosomal storage disorder Gaucher’s disease (GD), are the strongest genetic risk factor for Parkinson’s disease (PD) known to date. Here we generate induced pluripotent stem cells from subjects with GD and PD harbouring GBA1 mutations, and differentiate them into midbrain dopaminergic neurons followed by enrichment using fluorescence-activated cell sorting. Neurons show a reduction in glucocerebrosidase activity and protein levels, increase in glucosylceramide and α-synuclein levels as well as autophagic and lysosomal defects. Quantitative proteomic profiling reveals an increase of the neuronal calcium-binding protein 2 (NECAB2) in diseased neurons. Mutant neurons show a dysregulation of calcium homeostasis and increased vulnerability to stress responses involving elevation of cytosolic calcium. Importantly, correction of the mutations rescues such pathological phenotypes. These findings provide evidence for a link between GBA1 mutations and complex changes in the autophagic/lysosomal system and intracellular calcium homeostasis, which underlie vulnerability to neurodegeneration. Parkinson’s disease (PD) is the second most common neurodegenerative disorder, with >1% of the population over 65 years of age affected and >4% affected by the age of 85 years. Several clues to understanding disease pathogenesis come from mutations in genes, which have been linked to familial forms of PD or identified as risk factors. Among these, heterozygous mutations in the acid β-glucocerebrosidase ( GBA1 ) gene, which encodes the lysosomal enzyme β-glucocerebrosidase (GCase), have been linked to a higher risk of developing PD and other synucleinopathies [1] , [2] . GCase is a lysosomal enzyme that catalyses the hydrolysis of glucosylceramide (Glc-Cer) to ceramide and glucose. Homozygous mutations of GBA1 are responsible for Gaucher’s disease (GD), which is the most prevalent lysosomal storage disorder, characterized by decreased activity of GCase and subsequent accumulation of Glc-Cer in several organs including the brain. Different clinical forms are described depending on the absence (non-neuronopathic forms, GD type 1) or presence (neuronopathic forms, GD type 2 and 3) of neurological symptoms. GD type 1 is the most common type and is often associated with PD and parkinsonism, thus challenging such classification [3] . To date, over 300 mutations have been identified in GBA1 and linked to GD. In recent years, GD and PD have been connected on account of the clinical observation of parkinsonism and Lewy Body (LB) pathology in patients with GD [3] . Compared with the general population, patients with GD type 1 have a 20-fold increased lifetime risk of developing parkinsonism [4] , whereas individuals carrying heterozygous GBA1 mutations have a five times greater risk of developing PD than non-carrier individuals [1] . The pathological mechanisms through which the mutant enzyme causes PD still remain elusive and both gain- and loss-of-function theories have been postulated. Such hypotheses are not mutually exclusive and include increased α-synuclein (α-syn) protein aggregation, sphingolipid accumulation and impaired trafficking as potential mechanisms involved in the pathogenesis of neurodegeneration [5] , [6] . Recent progress in the induced pluripotent stem cell (iPSC) technology has allowed the generation of functional dopaminergic (DA) neurons from familial and sporadic PD subjects [7] , [8] , [9] , offering a unique opportunity to study the role of genetic mutations and risk factors in the pathogenesis of PD. Neurons from PD patients carrying heterozygous GBA1 mutations have not yet been generated, and it is unknown whether such cells recapitulate the pathological phenotypes observed in vivo . In this study, we demonstrate that iPSC-derived neurons from GD and PD individuals carrying GBA1 mutations display relevant disease phenotypes, including a significant reduction of GCase enzymatic activity and protein levels as well as increased levels of α-syn and Glc-Cer. Furthermore, mutant neurons show defects in the autophagic/lysosomal system and impaired intracellular calcium homeostasis. Importantly, such phenotypes are reverted upon gene correction, thus supporting a direct link between GBA1 mutations and disease-relevant phenotypes. 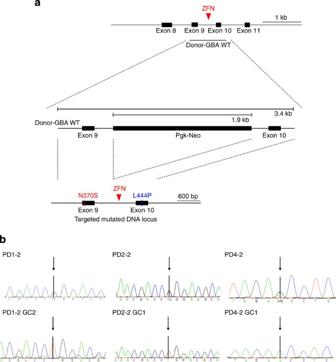Figure 1: Gene correction of GBA-PD iPSCs. (a) Structure of theGBA1gene on chromosome 1 and schematic overview of gene correction using ZFNs. Black boxes represent exons. (b) Mutated and gene-corrected (GC) iPSCs after sequencing (upper lanes: iPSCs with heterozygous mutations; lower lanes: iPSCs with homozygous wt-GBA1sequences as indicated by arrows). Generation of iPSCs and isogenic gene-corrected controls Skin fibroblasts were obtained from two healthy controls, four PD patients carrying heterozygous GBA1 mutations (RecNcil/wt; L444P/wt; N370S/wt) and four GD patients (type 1: N370S/N370S; type 3: L444P/L444P) ( Supplementary Table 1 ). Fibroblasts were reprogrammed by transduction with SOX2, OCT4, KLF4 and c-MYC retroviruses. 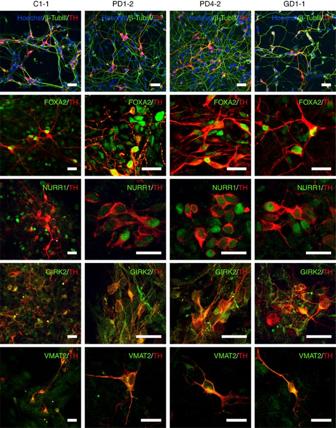Figure 2: Differentiation of iPSCs into mDA neurons. Immunostaining of indicated differentiated iPSC cultures at DIV65. Cells were stained for TH (red) and β-TubIII, FOXA2, NURR1, GIRK2 and VMAT2 (all green). Cell nuclei were counterstained with Hoechst (blue). (Bars, 20 μm). After 4 to 5 weeks, iPSC colonies were isolated and further characterized ( Supplementary Table 2 ). All generated iPSCs showed human embryonic stem cell (hESC)-like morphology and expressed alkaline phosphatase and the pluripotency markers SSEA4, TRA-1-81, TRA-1-60, OCT4, NANOG and LIN28 ( Supplementary Figs 1 and 2a ). iPSCs were genetically matched with their parental cells by PCR-based DNA fingerprinting analysis, maintained euploid karyotypes over several passages in vitro and showed effective silencing of the exogenous transgenes and upregulation of endogenous hESC markers ( Supplementary Fig. 2b–d ). All lines tested were efficiently differentiated to mesoderm, endoderm and ectoderm in vitro ( Supplementary Fig. 3a ) and formed teratomas consisting of the three germ layers when injected into the kidney capsule and testis of immune-compromised mice ( Supplementary Fig. 3b ). Correction of GBA1 mutations in iPSCs was performed by zinc-finger nuclease (ZFN)-mediated homologous recombination. Three iPSC lines (PD1-2, PD2-2 and PD4-2) were selected for gene-targeting experiments. iPSCs were nucleofected with ZFNs, which were designed to introduce a double-strand brake adjacent to the N370S and L444P mutations, along with a wild-type (wt)-GBA1 construct harbouring a neomycin resistance cassette ( Fig. 1a ). Single resistant colonies were selected, and corrected sequences at the mutation site were confirmed by DNA and RNA sequencing ( Fig. 1b ). Karyotype analysis revealed that no translocation had occurred in the clones after ZFN-mediated insertion. Figure 1: Gene correction of GBA-PD iPSCs. ( a ) Structure of the GBA1 gene on chromosome 1 and schematic overview of gene correction using ZFNs. Black boxes represent exons. ( b ) Mutated and gene-corrected (GC) iPSCs after sequencing (upper lanes: iPSCs with heterozygous mutations; lower lanes: iPSCs with homozygous wt- GBA1 sequences as indicated by arrows). Full size image Differentiation of iPSCs to mDA neurons iPSCs from controls, GBA-PD and GD subjects were differentiated to mDA neurons by using a floor-plate-based neural differentiation protocol [10] . This early neural patterning protocol induces 70% FOXA2 + /OTX2 + floor plate precursors by day 11 (ref. 10 and Supplementary Fig. 4 ). By day 40, all iPSC lines generated β-TubIII + neurons and cells expressing tyrosine hydroxylase (TH). At DIV 65, 15–20% of the cells were TH + and co-expressed markers of mDA phenotype (FOXA2, NURR1, GIRK2, VMAT2) ( Fig. 2 ). No significant differences in differentiation potential were observed among control, GBA-PD, gene-corrected and GD lines ( Supplementary Fig. 5a ). Differentiated neurons showed a punctate staining of synapsin 1, indicating the presence of synaptically mature neurons ( Supplementary Fig. 5b ). Figure 2: Differentiation of iPSCs into mDA neurons. Immunostaining of indicated differentiated iPSC cultures at DIV65. Cells were stained for TH (red) and β-TubIII, FOXA2, NURR1, GIRK2 and VMAT2 (all green). Cell nuclei were counterstained with Hoechst (blue). (Bars, 20 μm). Full size image Enrichment of neuronal populations from differentiated iPSCs To enrich neuronal populations from differentiated iPSC cultures, we included a neuronal cell isolation step using fluorescence-activated cell sorting (FACS) [11] , [12] , [13] , [14] . At DIV 65–70, differentiated neurons from iPSCs were purified based on a surface marker code of CD24 high CD29 − CD184 − CD44 − CD15 − ( Fig. 3a ). Analysis of post-FACS cell cultures revealed highly enriched neuronal populations (6.1-fold enrichment compared with unsorted cells), which expressed mature DA neuronal markers and could be kept in vitro for 3 weeks after sorting ( Fig. 3b,c and Supplementary Fig. 6 ). Whole-cell patch clamp recordings showed that single neurons were able to fire action potentials (AP) repetitively. Importantly, around 50% of the patched neurons derived from iPSCs showed spontaneous firing activity ( Supplementary Fig. 7a ), whereas in 93% of the recorded cells AP could be elicited by current injections into the soma ( Supplementary Fig. 7b ). The mean resting membrane potential of all recorded neurons was −53.1±1.5 mV. In addition, recorded cells showed sodium and potassium currents ( Supplementary Fig. 7c ). Importantly, differentiated neuronal cultures released DA ( Supplementary Fig. 7d ). 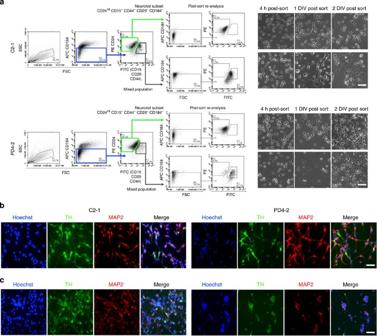Figure 3: FACS enriches for neuronal populations. (a) Gating strategy used for neuronal cell sorting. Live cells as determined by FSC/SSC gating were selected for CD184-APC-negative/low surface expression and subsequently separated for CD24-PE versus CD15/CD29/CD44 expression, detected in the FITC channel as indicated in the dot plots. Post-sort reanalysis shows representative samples of both fractions immediately after FACS enrichment, which were then plated for comparativein vitroanalysis (phase contrast images. Bars, 50 μm). (b,c) Immunocytochemistry at DIV2 post-sort for TH (green) and the neuronal marker MAP2 (red) performed on the neuronal (b) and mixed (c) populations of a representative control and GBA-PD line. Nuclei were counterstained with Hoechst (blue). FACS enriches for both TH and neuronal marker positivity in the neuronal population compared with the non-neuronal population. (Bars, 50 μm.) Figure 3: FACS enriches for neuronal populations. ( a ) Gating strategy used for neuronal cell sorting. Live cells as determined by FSC/SSC gating were selected for CD184-APC-negative/low surface expression and subsequently separated for CD24-PE versus CD15/CD29/CD44 expression, detected in the FITC channel as indicated in the dot plots. Post-sort reanalysis shows representative samples of both fractions immediately after FACS enrichment, which were then plated for comparative in vitro analysis (phase contrast images. Bars, 50 μm). ( b , c ) Immunocytochemistry at DIV2 post-sort for TH (green) and the neuronal marker MAP2 (red) performed on the neuronal ( b ) and mixed ( c ) populations of a representative control and GBA-PD line. Nuclei were counterstained with Hoechst (blue). FACS enriches for both TH and neuronal marker positivity in the neuronal population compared with the non-neuronal population. (Bars, 50 μm.) Full size image The polysialoganglioside content of iPSC-derived neurons Gangliosides are sphingolipids (GSL) particularly abundant in the neuronal plasma membrane playing an important role in the pathogenesis of neurological disorders. With respect to synucleinopathies, alterations in the neuronal GSL composition cause impaired α-syn membrane binding and enhanced aggregation in the cytoplasm [15] . To study the link between GCase and α-syn and to investigate the pathogenesis of neurodegeneration in sphingolipidoses, it is therefore crucial to utilize cell models that resemble the GSL composition and pattern of adult human brain. The content and pattern of gangliosides markedly change during brain development [16] and the ganglioside concentration is ~\n10 times higher in the brain than in other organs [17] . The total brain ganglioside content is very low at the embryonic and fetal stage and then increases several folds with a shift from gangliosides of the Lac series, GM3 and GD3, to monosialo-, during development, and polysialo-species in the adult brain [16] , [17] . The GSL content and pattern are therefore useful markers to follow neural development both in vivo and in vitro [18] , [19] . To investigate whether iPSCs recapitulate such developmental changes during in vitro differentiation and whether iPSC-derived neurons have the GSL composition of developmentally mature neurons, we metabolically labelled gangliosides by feeding fibroblasts, iPSCs and iPSC-derived neurons (before and after FACS enrichment) from control, GBA-PD and GD type 3 subjects with isotopically tritium labelled [1– 3 H]sphingosine [19] . After a 48-hour chase, gangliosides were purified from the total lipid extract, separated by HPTLC and analysed by radio-imaging [20] . As expected, the ganglioside pattern of fibroblasts was characterized by the presence of GM3 and a minor quantity of GD3 ( Fig. 4a ). Minor differences in the ganglioside pattern and in the GM3/GD3 ratio among fibroblast cell lines were detected ( Fig. 4a ), which have been described to be age and patient specific [21] . In iPSC cultures, GM3 still represented the main ganglioside, but low amounts of GM2, GM1 and GD1a components were identified ( Fig. 4a ). By contrast, differentiated iPSCs contained all the polysialogangliosides found in the CNS, even though high levels of GM3 and GD3 were still present [16] ( Fig. 4a and Supplementary Fig. 8 ). After FACS enrichment, the levels of GD3 and GM3 were found to be significantly reduced compared with the total GSL composition and the levels of GM1, GD1a, GD1b and GT1b were in a percentage distribution similar to that found in the adult human and rodent brain ( Fig. 4a and Supplementary Fig. 9 ) [22] . Importantly, the total ganglioside content in FACS-enriched iPSC-derived neurons was about 10 times higher than that in fibroblasts: the radioactivity associated with gangliosides ranged from 41,250 to 57,500 dpm mg −1 cell protein in fibroblasts (control, GD and GBA-PD) and from 330,650 to 415,000 dpm mg −1 cell protein in sorted neurons. 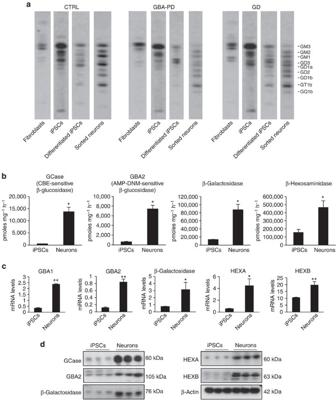Figure 4: Ganglioside and glycohydrolase changes during human iPSC differentiation recapitulate human brain development. (a) Ganglioside composition of human fibroblasts, iPSCs, differentiated iPSCs and enriched iPSC-derived neurons (after FACS) from control (line C1-1), GBA-PD (line PD1-1) and GD (line GD1-1) subjects. Cell lipids were metabolically labelled with [1-3H]sphingosine and visualized by digital autoradiography. (b) Activities of glycohydrolases (GCase, GBA2, β-galactosidase, β-hexosaminidase) in control iPSCs and iPSC-derived enriched neurons at DIV65. Enzyme activities are expressed as pmoles mg−1h−1. Data are represented as mean+s.d.; experiments were independently repeated three times in triplicate. *P<0.01; Student’st-test. (c) GBA1, GBA2, β-galactosidase and HEXA and HEXB gene expression levels in control iPSCs and iPSC-derived enriched neurons at DIV65. Data are represented as mean+s.d.; experiments were independently repeated three times in triplicate. *P<0.05; **P<0.01, Student’st-test. (d) Representative western blots showing GCase, GBA2, β-galactosidase and HEXA and HEXB protein levels in control iPSCs and corresponding iPSC-derived neurons (DIV65). Figure 4: Ganglioside and glycohydrolase changes during human iPSC differentiation recapitulate human brain development. ( a ) Ganglioside composition of human fibroblasts, iPSCs, differentiated iPSCs and enriched iPSC-derived neurons (after FACS) from control (line C1-1), GBA-PD (line PD1-1) and GD (line GD1-1) subjects. Cell lipids were metabolically labelled with [1- 3 H]sphingosine and visualized by digital autoradiography. ( b ) Activities of glycohydrolases (GCase, GBA2, β-galactosidase, β-hexosaminidase) in control iPSCs and iPSC-derived enriched neurons at DIV65. Enzyme activities are expressed as pmoles mg −1 h −1 . Data are represented as mean+s.d. ; experiments were independently repeated three times in triplicate. * P <0.01; Student’s t -test. ( c ) GBA1, GBA2, β-galactosidase and HEXA and HEXB gene expression levels in control iPSCs and iPSC-derived enriched neurons at DIV65. Data are represented as mean+s.d. ; experiments were independently repeated three times in triplicate. * P <0.05; ** P <0.01, Student’s t -test. ( d ) Representative western blots showing GCase, GBA2, β-galactosidase and HEXA and HEXB protein levels in control iPSCs and corresponding iPSC-derived neurons (DIV65). Full size image Glycohydrolases in human iPSCs and enriched neurons The developmental changes of GSL content and patterns can be largely attributed to switches in the expression and activity of several enzymes involved in their synthesis and catabolism [16] . We therefore investigated the activities of enzymes involved in the catabolic pathway of GSL during human iPSC differentiation. Control iPSCs were differentiated for 65–70 days in vitro , neurons enriched by FACS and the activities of the main hydrolases involved in the metabolism of glycoconjugates (conduritol B epoxide (CBE)-sensitive β-glucosidase, non-lysosomal β-glucosyl ceramidase (GBA2), β-galactosidase and β-hexosaminidase) were investigated. Two different cellular compartment-specific β-glucosidase activities were analysed: the lysosomal β-glucocerebrosidase GCase and the non-lysosomal beta-glucosyl ceramidase GBA2 (ref. 23 ). By using CBE, a specific inhibitor of GCase, it was possible to evaluate the activity associated with GBA2, whereas, by application of the specific inhibitor N -(5-adamantane-1-yl-methoxy-pentyl)-deoxynojirimycin (AMP-DNM) [24] , it was possible to determine the β-glucosidase activity due to GCase. We found that the activity of all tested enzymes was significantly increased in iPSC-derived neurons compared with iPSCs and fibroblasts, suggesting an important role of such enzymes in differentiation and maintenance of GSL composition in neurons ( Fig. 4b and Supplementary Fig. 10a ). Quantitative RT-PCR and immunoblot revealed an increase in GBA1, GBA2, β-galactosidase and β-hexosaminidase mRNA and protein levels in differentiated cultures compared with iPSCs ( Fig. 4c,d ). Increased Glc-Cer and α-syn levels in GBA1 mutant neurons Recent studies using iPSC-derived neurons from GD patients showed that DA neurons accumulate glycosphingolipids [25] , [26] . To examine whether neurons from PD patients carrying heterozygous GBA1 mutations also display such phenotypes, we carried out liquid chromatography (LC) and tandem mass spectrometry (MS) (LC-MS/MS) analysis on differentiated iPSCs from controls, GBA-PD and GD patients. Both homozygous and heterozygous GBA1 mutant iPSC-derived neurons showed elevated levels of Glc-Cer compared with control cells ( Fig. 5a ). Importantly, gene-corrected isogenic controls showed reduced Glc-Cer levels compared with the parental lines ( Fig. 5a ). 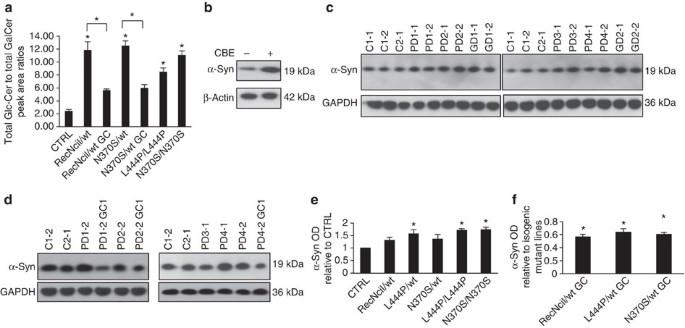Figure 5: Glc-Cer and α-syn levels are increased in GBA-PD and GD iPSC-derived neurons. (a) LC-MS/MS analysis showing the level of Glc-Cer in control, GBA-PD, isogenic controls and GD iPSC-derived neurons. Data are represented as mean+s.d.;n=3, *P<0.01, One-way ANOVA. (b) Control iPSCs (line C1-1) were differentiated for 65 days and exposed to the GCase inhibitor CBE (25 μM) for 48 h. Representative western blot showing increased levels of α-syn in CBE-treated iPSC-derived neurons compared to untreated neurons. (c,d) Representative western blots showing the protein levels of α-syn in control, GBA-PD, gene-corrected isogenic controls and GD iPSC-derived neurons. (e) Optical densities of α-syn bands normalized by the averaged value of GAPDH and expressed as a percentage of the control (CTRL) line value. Data are represented as mean+s.d.; experiments were independently repeated five times. *P<0.01, one-way ANOVA. (f) Average α-syn protein levels normalized by the averaged value of GAPDH and expressed as a percentage of the respective isogenic mutant lines. Data are represented as mean+s.d.; experiments were independently repeated five times. *P<0.01, Student’st-test. Figure 5: Glc-Cer and α-syn levels are increased in GBA-PD and GD iPSC-derived neurons. ( a ) LC-MS/MS analysis showing the level of Glc-Cer in control, GBA-PD, isogenic controls and GD iPSC-derived neurons. Data are represented as mean+s.d. ; n =3, * P <0.01, One-way ANOVA. ( b ) Control iPSCs (line C1-1) were differentiated for 65 days and exposed to the GCase inhibitor CBE (25 μM) for 48 h. Representative western blot showing increased levels of α-syn in CBE-treated iPSC-derived neurons compared to untreated neurons. ( c , d ) Representative western blots showing the protein levels of α-syn in control, GBA-PD, gene-corrected isogenic controls and GD iPSC-derived neurons. ( e ) Optical densities of α-syn bands normalized by the averaged value of GAPDH and expressed as a percentage of the control (CTRL) line value. Data are represented as mean+s.d. ; experiments were independently repeated five times. * P <0.01, one-way ANOVA. ( f ) Average α-syn protein levels normalized by the averaged value of GAPDH and expressed as a percentage of the respective isogenic mutant lines. Data are represented as mean+s.d. ; experiments were independently repeated five times. * P <0.01, Student’s t -test. Full size image A direct link between GCase and α-syn accumulation has previously been shown [25] , [27] , [28] . However, it has not yet been investigated whether heterozygous GBA1 mutations are linked to increased levels of α-syn. We therefore sought to examine the effects of GBA1 mutations on α-syn accumulation in differentiated iPSCs. First, we examined the effect of loss of GCase activity in control iPSC-derived neurons. We found that CBE treatment induced an increase in α-syn protein levels in control iPSC-derived neurons ( Fig. 5b ). Next, iPSCs from controls, GBA-PD and GD subjects were differentiated to mDA neurons, and α-syn levels were measured by western blot. A significant increase in α-syn protein levels was found in GBA-PD neurons carrying the L444P allele and in GD neurons compared with controls ( Fig. 5c,e ). It is known that differences in expression levels of α-syn are influenced by individual genetic background, which could explain the high variability of α-syn expression in the general population [29] . Thus, we measured α-syn levels in neuronal cultures from GBA-PD iPSCs and corresponding isogenic gene-corrected controls. Interestingly, we found a significant reduction in α-syn levels in all gene-corrected neurons (RecNcil, L444P, N370S) compared with their parental lines ( Fig. 5d,f ). Reduced GCase in GBA1 mutant neurons The GCase activity was significantly reduced in GBA-PD and GD fibroblasts compared with healthy control cells ( Supplementary Fig. 11 ). Next, control, GBA-PD, isogenic gene-corrected controls and GD iPSCs were differentiated for 65 days and neuronal cultures were enriched by FACS. We found that the GCase enzymatic activity was significantly reduced in GBA-PD and GD neurons compared with controls ( Fig. 6a ). Importantly, isogenic gene-corrected lines showed a significantly higher average of enzymatic activity compared with non-corrected lines ( Fig. 6a ). Quantitative analysis of intracellular GCase protein levels in cells of different patients by western-blotting revealed that protein levels of the enzyme were also reduced in GBA-PD and GD patients compared with control individuals ( Fig. 6b,c ). ZFN-mediated gene correction rescued the levels of GCase ( Fig. 6b,c ). 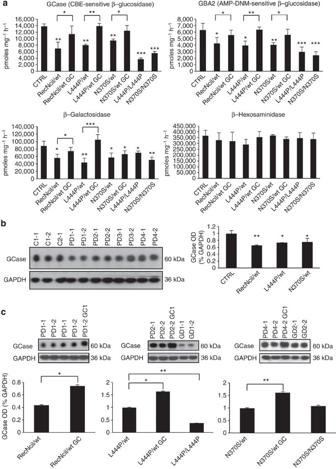Figure 6: GBA-PD and GD iPSC-derived neurons show decreased glycohydrolase enzyme activities and protein levels. (a) Glycohydrolase enzyme activities (GCase, GBA2, β-galactosidase, β-hexosaminidase) were measured in enriched neurons from control, GBA-PD, isogenic gene-corrected control and GD iPSC-derived neurons at DIV65. Enzyme activities are expressed as pmoles mg−1h−1. Data are represented as mean+s.d.; experiments were independently repeated three times in triplicate. *P<0.05; **P<0.01; ***P<0.001 compared with controls, one-way ANOVA. (b,c) Representative western blots of GCase protein levels in control, GBA-PD, corresponding gene-corrected and GD iPSC-derived neurons. Data are represented as mean+s.d.; experiments were independently repeated three times. *P<0.05; **P<0.01, one-way ANOVA and Student’st-test. Figure 6: GBA-PD and GD iPSC-derived neurons show decreased glycohydrolase enzyme activities and protein levels. ( a ) Glycohydrolase enzyme activities (GCase, GBA2, β-galactosidase, β-hexosaminidase) were measured in enriched neurons from control, GBA-PD, isogenic gene-corrected control and GD iPSC-derived neurons at DIV65. Enzyme activities are expressed as pmoles mg −1 h −1 . Data are represented as mean+s.d. ; experiments were independently repeated three times in triplicate. * P <0.05; ** P <0.01; *** P <0.001 compared with controls, one-way ANOVA. ( b , c ) Representative western blots of GCase protein levels in control, GBA-PD, corresponding gene-corrected and GD iPSC-derived neurons. Data are represented as mean+s.d. ; experiments were independently repeated three times. * P <0.05; ** P <0.01, one-way ANOVA and Student’s t -test. Full size image Decreased glycohydrolase activities in GBA1 mutant neurons We next analysed the activity of additional glycohydrolases in iPSC-derived neurons from controls, GBA-PD, isogenic gene-corrected controls and GD subjects. Activity levels of the lysosomal enzymes β-galactosidase and β-hexosaminidase, as well as the activity of the non-lysosomal β-glucosylceramidase GBA2, were examined in differentiated iPSC-neurons after FACS enrichment. Our analysis revealed a significant decrease in the activity of GBA2 and β-galactosidase in GBA-PD and GD neurons compared with healthy controls, whereas activity levels of β-hexosaminidase remained unchanged ( Fig. 6a ). Interestingly, gene correction rescued such changes in RecNcil- and L444P-associated PD lines ( Fig. 6a ). Gene expression levels of GBA2 and β-galactosidase in patient neurons were unchanged compared with control neurons ( Supplementary Fig. 10b ). An increase in the activity of GBA2, β-hexosaminidase and β-galactosidase has recently been described in GD fibroblasts and leukocytes [30] , [31] . We therefore examined the enzyme activities in respective fibroblast lines and found a significant increase in GBA2 activity in GBA-PD (L444P/wt) and GD (L444P/L444P) fibroblasts, while GD fibroblasts (L444P/L444P) showed in addition a significant increase in β-galactosidase activity compared with controls ( Supplementary Fig. 11 ). Glycohydrolase activities in the CSF of GBA-PD patients Recent studies showed that GCase activity is lower in the cerebrospinal fluid (CSF) and brain samples of patients with PD or dementia with LB than that in healthy individuals [32] , [33] , [34] . To determine whether changes in iPSC-derived neurons were accompanied by changes in the glycohydrolase enzymatic activity in the CSF, we measured the activity of several glycohydrolases (GCase, GBA2, β-galactosidase, β-hexosaminidase, α-fucosidase, α- and β-mannosidase) in the CSF of PD patients carrying heterozygous RecNcil, L444P or N370S GBA1 mutations, idiopathic PD patients as well as age-matched unaffected controls. Enzyme activity levels were normalized against total protein levels. The CSF of patients used for iPSC generation in this study was included in the analysis. No significant differences between idiopathic PD patients and controls were observed for all tested enzymes ( Fig. 7 ); however, in GBA-PD patients the activities of GCase, GBA2 and β-galactosidase were significantly reduced compared with unaffected controls ( Fig. 7 ). In addition, we found a significant reduction in the enzyme activity of GCase, GBA2, α- and β-mannosidase in GBA-PD patients compared with idiopathic PD patients ( Fig. 7 ). 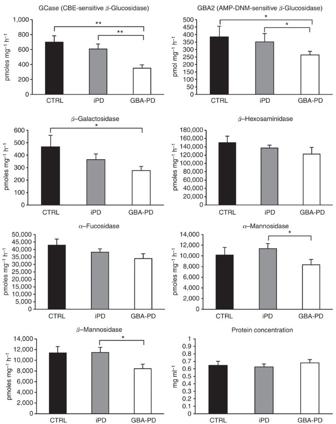Figure 7: Glycohydrolase enzyme activities in the CSF of unaffected individuals, GBA-PD and idiopathic PD patients. CSF glycohydrolase activities were measured in patients with idiopathic PD (iPD), GBA-PD patients and age-matched unaffected individuals (CTRL). Enzyme activities were normalized to total protein concentrations and expressed as pmoles mg−1h−1. Data are represented as mean+s.e.m.; CTRL,n=14; iPD,n=15; GBA-PD,n=15. Experiments were performed in triplicate. *P<0.05; **P<0.01, Mann–WhitneyUtest. Figure 7: Glycohydrolase enzyme activities in the CSF of unaffected individuals, GBA-PD and idiopathic PD patients. CSF glycohydrolase activities were measured in patients with idiopathic PD (iPD), GBA-PD patients and age-matched unaffected individuals (CTRL). Enzyme activities were normalized to total protein concentrations and expressed as pmoles mg −1 h −1 . Data are represented as mean+s.e.m. ; CTRL, n =14; iPD, n =15; GBA-PD, n =15. Experiments were performed in triplicate. * P <0.05; ** P <0.01, Mann–Whitney U test. Full size image Lysosomal and autophagic defects in GBA1 mutant neurons To extend these findings, we analysed the autophagic/lysosomal machinery in GBA1 mutant neurons. Immunofluorescent staining for LAMP1, a lysosomal marker, revealed a significant increase in number and size of LAMP1 + particles in patient iPSC-derived neurons compared with healthy individuals, suggesting an accumulation of lysosomes ( Fig. 8a,b and Supplementary Fig. 12a ). To examine macroautophagy, we first investigated the autophagosome content by immunostaining for endogenous light chain type 3 protein (LC3), a marker of autophagosomes. Our analysis revealed a significant increase of LC3 + vesicles in GBA-PD and GD neurons compared with control neurons ( Supplementary Fig. 12b,d ). These results were confirmed by immunoblot, which showed an increase in basal levels of LC3-II in GBA-PD and GD-derived neurons ( Fig. 8c,d ). Inhibition of lysosomal degradation by leupeptin and ammonium chloride (NH 4 Cl) revealed that the autophagic flux was significantly reduced in GBA-PD and GD neurons ( Fig. 8e ). To examine autophagosome-lysosome fusion, we assessed the co-localization of LC3 and LAMP1 markers in iPSC-derived neurons. We observed a decreased degree of co-localization between LC3 + vacuoles and LAMP1 + vacuoles in GBA-PD and GD neurons, which suggests an impaired autophagosome-lysosome fusion in GBA1 mutant neurons. ( Supplementary Fig. 12c,e ). 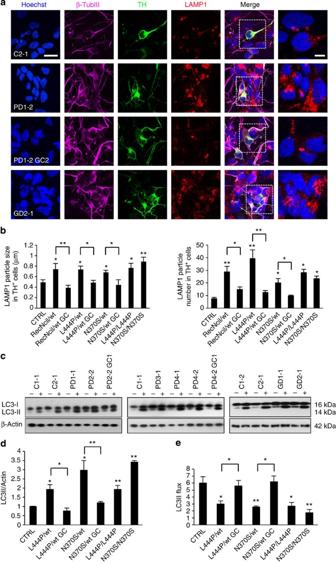Figure 8: GBA-PD and GD iPSC-derived neurons show alterations in the autophagic/lysosomal system. (a) Immunostaining of differentiated iPSC cultures at DIV65 under basal conditions. Cells were stained for TH (green), β-TubIII (magenta) and LAMP1 (red). Cell nuclei were counterstained with Hoechst (blue). High magnification insets are shown in the right lane. (Bars, 20 μm and 10 μm in the insets.) (b) Average size and number of LAMP1+particles in TH+neurons were quantified by ImageJ. Data are represented as mean+s.e.m.; experiments were independently repeated three times in triplicate. *P<0.01, **P<0.001, one-way ANOVA. (c) Western blot analysis for LC3 in iPSC-derived neuronal cultures at DIV65, untreated (−) or treated with 200 μM leupeptin and 20 mM NH4Cl for 4 h (+). (d) Quantification of the basal levels of LC3-II relative to β-actin. Data are represented as mean+s.e.m.; experiments were independently repeated three times. *P<0.01; **P<0.001, one-way ANOVA. (e) Quantification of LC3 flux normalized to actin. Data are represented as mean+s.e.m.; experiments were independently repeated three times in triplicate. *P<0.01; **P<0.001, one-way ANOVA. Figure 8: GBA-PD and GD iPSC-derived neurons show alterations in the autophagic/lysosomal system. ( a ) Immunostaining of differentiated iPSC cultures at DIV65 under basal conditions. Cells were stained for TH (green), β-TubIII (magenta) and LAMP1 (red). Cell nuclei were counterstained with Hoechst (blue). High magnification insets are shown in the right lane. (Bars, 20 μm and 10 μm in the insets.) ( b ) Average size and number of LAMP1 + particles in TH + neurons were quantified by ImageJ. Data are represented as mean+s.e.m. ; experiments were independently repeated three times in triplicate. * P <0.01, ** P <0.001, one-way ANOVA. ( c ) Western blot analysis for LC3 in iPSC-derived neuronal cultures at DIV65, untreated (−) or treated with 200 μM leupeptin and 20 mM NH 4 Cl for 4 h (+). ( d ) Quantification of the basal levels of LC3-II relative to β-actin. Data are represented as mean+s.e.m. ; experiments were independently repeated three times. * P <0.01; ** P <0.001, one-way ANOVA. ( e ) Quantification of LC3 flux normalized to actin. Data are represented as mean+s.e.m. ; experiments were independently repeated three times in triplicate. * P <0.01; ** P <0.001, one-way ANOVA. Full size image Impaired calcium homeostasis in GBA1 mutant neurons We next used quantitative mass spectrometry (MS)-based proteomics to search for proteins whose levels are affected by GBA1 mutations in iPSC-derived neurons. Two independent iPSC lines harbouring the L444P allele and three independent control lines were differentiated and enriched by FACS. We extracted proteins and performed quantitative proteomic profiling by isotopic labelling (tandem mass tag, TMT) and MS analysis ( Table 1 , Supplementary Fig. 13a,b and Supplementary Data 1 ). In total, 7,069 proteins were identified from enriched neurons at a protein false-discovery rate (FDR) <1%. We calculated the differences in protein abundances between GBA-PD neurons and control lines, tested for statistical significance by t -test analysis and filtered for proteins whose levels changed by at least 1.2-fold ( Table 1 ). To validate the MS proteomic data, immunoblotting of selected proteins was performed on three independent differentiated iPSC cultures ( Supplementary Fig. 13a ). Among the differentially expressed proteins, we found that the neuronal calcium-binding protein 2 (NECAB2) was significantly upregulated (1.9-fold) in lines harbouring the L444P allele ( Table 1 and Supplementary Fig. 13a ). Calcium-induced excitotoxicity plays a key role in the pathogenesis of several neurodegenerative diseases including PD [35] . To further investigate the potential role of calcium in the vulnerability of neurons harbouring GBA1 mutations, we examined calcium homeostasis using the calcium dye Fura-2 acetoxymethyl ester and compared calcium levels in control and diseased neurons. Interestingly, we found a significant increase in the basal calcium levels in GBA-PD and GD iPSC-derived neurons compared with controls ( Fig. 9a ). We therefore investigated the effects of caffeine, a RyR agonist that increases the calcium release from the calcium-sensitive internal stores, namely the endoplasmic reticulum (ER), into the cytoplasm. Caffeine induced an increase in cytosolic calcium, which was significantly greater in GBA-PD (L444P/wt) and GD neurons compared with control neurons ( Fig. 9b and Supplementary Fig. 14a ). Although we also found a consistent trend for increased calcium levels in GBA-PD (RecNcil/wt) neurons, this increase was not statistically significant ( Fig. 9b ). However, intracellular calcium levels in response to caffeine stimulation were comparable between isogenic gene-corrected neurons (both L444P/wt and RecNcil/wt) and control neurons ( Fig. 9b and Supplementary Fig. 14a ), suggesting a role of GBA1 mutations in regulating intracellular calcium concentration. Our data therefore indicate that RyR-mediated calcium release is increased in the presence of GBA1 mutations. We next examined the vulnerability of mutant neurons to ER stress responses by application of either A23187 (0–5 μM), a calcium ionophore that induces ER stress by increasing the cytosolic calcium concentration, or rotenone (0–200 nM), an inhibitor of complex I of the mitochondrial electron transport chain, which induces mitochondrial ROS production and elevation of intracellular levels of calcium [36] , [37] . Neuronal vulnerability was assessed by measuring cellular release of lactate dehydrogenase (LDH). Our results show that neurons carrying GBA1 mutations were more sensitive to A23187 (1–2.5 μM) and rotenone (50–200 nM) than control cells ( Fig. 9c and Supplementary Fig. 15a ). Immunocytochemistry and cell counts of TH + cells confirmed the increased vulnerability of mutant neurons ( Fig. 9d and Supplementary Fig. 15b ). Importantly, such a phenotype was rescued by gene correction. To gain insight into the functional role of NECAB2, we knocked down NECAB2 in iPSC-derived neurons using lentiviral-mediated short hairpin RNA (shRNA). The gene expression and protein levels of NECAB2 were reduced by ~\n80% in knocked down iPSC-derived neurons ( Fig. 9e,f ). To further examine the functional role of NECAB2, iPSC-derived neurons were exposed to A23187 and neurotoxicity was assessed by immunostaining for TH. We found that knockdown of NECAB2 resulted in a statistically significant increase of calcium-mediated neurotoxicity ( Fig. 9g,h ). In addition, calcium-imaging experiments revealed an increase in caffeine-induced cytosolic calcium levels after NECAB2 knockdown ( Supplementary Fig. 14b ). Table 1 Identification of proteins with changed expression levels in iPSC-derived enriched neurons carrying GBA1 mutations. 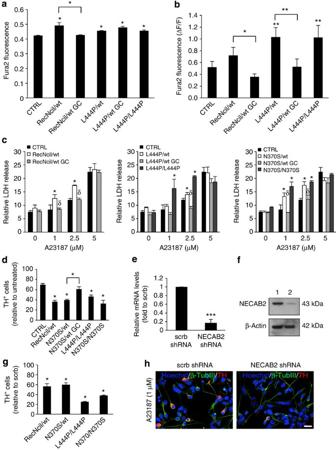Figure 9: Calcium homeostasis is dysregulated in GBA-PD and GD iPSC-derived neurons. (a) Cytosolic calcium levels were evaluated in iPSC-derived neurons at basal conditions by measuring the 340/380 nm ratio of Fura-2 acetoxymethyl ester. Data are represented as mean+s.e.m.; experiments were independently repeated three times in triplicate. *P<0.01; Student’st-test. (Number of cells analysed: CTRL,n=58; RecNcil/wt,n=36; RecNcil/wt GC,n=107; L444P/wt,n=82; L444P/wt GC,n=33; L444P/L444P,n=62). (b) Caffeine (10 mM) was applied to iPSC-derived neurons, and the peak cytosolic calcium concentration was measured as a change in Fura-2 fluorescence. Data are represented as mean+s.e.m.; experiments were independently repeated three times in triplicate. *P<0.01; **P<0.001, Student’st-test. (Number of cells analysed: CTRL,n=58; RecNcil/wt,n=36; RecNcil/wt GC,n=107; L444P/wt,n=82; L444P/wt GC,n=33; L444P/L444P,n=62). (c) iPSC-derived neurons were treated with A23187 (0–5 μM) for 4 h and cytotoxicity was evaluated by released LDH activity. LDH release values were calculated as the percentage of untreated cells lysed by incubation with Triton X-100. Data are represented as mean+s.e.m.; experiments were independently repeated four times in triplicate. *P<0.05, one-way ANOVA, control lines versus mutated lines; δP<0.05, one-way ANOVA, mutated lines versus isogenic gene corrected controls. (d) Quantification of TH+cells treated with A23187 (1 μM) for 4 h expressed as a percentage of DMSO-treated controls. Data are represented as mean+s.d.; experiments were independently repeated three times in triplicate. *P<0.01, one-way ANOVA. (e) Knockdown efficiency of NECAB2 determined by qRT-PCR and normalized to scrambled non-targeting shRNA. Data are represented as mean+s.d.; experiments were independently repeated three times in triplicate. ***P<0.0001, Student’st-test. (f) Representative western blot for NECAB2 showing knockdown efficiency. 1, scrambled non-targeting shRNA; 2, NECAB2 shRNA. (g) Quantification of TH+cells in GBA-PD and GD iPSC-derived neuronal cultures infected with scrambled non-targeting shRNA or NECAB2 shRNA lentivirus and treated with A23187 (1 μM for 4 h). Values were calculated as a percentage of scrambled shRNA-treated cells. Data are represented as mean+s.e.m.; experiments were independently repeated three times in triplicate. *P<0.01, Student’st-test. (h) Representative images showing GBA-PD iPSC-derived DA neurons infected with scrambled non-targeting shRNA or NECAB2 shRNA lentivirus and treated with A23187 (1 μM for 4 h). Cells were stained for β-TubIII (green) and TH (red). Nuclei were counterstained with Hoechst (blue). (Bar, 20 μm.) Full size table Figure 9: Calcium homeostasis is dysregulated in GBA-PD and GD iPSC-derived neurons. ( a ) Cytosolic calcium levels were evaluated in iPSC-derived neurons at basal conditions by measuring the 340/380 nm ratio of Fura-2 acetoxymethyl ester. Data are represented as mean+s.e.m. ; experiments were independently repeated three times in triplicate. * P <0.01; Student’s t -test. (Number of cells analysed: CTRL, n =58; RecNcil/wt, n =36; RecNcil/wt GC, n =107; L444P/wt, n =82; L444P/wt GC, n =33; L444P/L444P, n =62). ( b ) Caffeine (10 mM) was applied to iPSC-derived neurons, and the peak cytosolic calcium concentration was measured as a change in Fura-2 fluorescence. Data are represented as mean+s.e.m. ; experiments were independently repeated three times in triplicate. * P <0.01; ** P <0.001, Student’s t -test. (Number of cells analysed: CTRL, n =58; RecNcil/wt, n =36; RecNcil/wt GC, n =107; L444P/wt, n =82; L444P/wt GC, n =33; L444P/L444P, n =62). ( c ) iPSC-derived neurons were treated with A23187 (0–5 μM) for 4 h and cytotoxicity was evaluated by released LDH activity. LDH release values were calculated as the percentage of untreated cells lysed by incubation with Triton X-100. Data are represented as mean+s.e.m. ; experiments were independently repeated four times in triplicate. * P <0.05, one-way ANOVA, control lines versus mutated lines; δ P <0.05, one-way ANOVA, mutated lines versus isogenic gene corrected controls. ( d ) Quantification of TH + cells treated with A23187 (1 μM) for 4 h expressed as a percentage of DMSO-treated controls. Data are represented as mean+s.d. ; experiments were independently repeated three times in triplicate. * P <0.01, one-way ANOVA. ( e ) Knockdown efficiency of NECAB2 determined by qRT-PCR and normalized to scrambled non-targeting shRNA. Data are represented as mean+s.d. ; experiments were independently repeated three times in triplicate. *** P <0.0001, Student’s t -test. ( f ) Representative western blot for NECAB2 showing knockdown efficiency. 1, scrambled non-targeting shRNA; 2, NECAB2 shRNA. ( g ) Quantification of TH + cells in GBA-PD and GD iPSC-derived neuronal cultures infected with scrambled non-targeting shRNA or NECAB2 shRNA lentivirus and treated with A23187 (1 μM for 4 h). Values were calculated as a percentage of scrambled shRNA-treated cells. Data are represented as mean+s.e.m. ; experiments were independently repeated three times in triplicate. * P <0.01, Student’s t -test. ( h ) Representative images showing GBA-PD iPSC-derived DA neurons infected with scrambled non-targeting shRNA or NECAB2 shRNA lentivirus and treated with A23187 (1 μM for 4 h). Cells were stained for β-TubIII (green) and TH (red). Nuclei were counterstained with Hoechst (blue). (Bar, 20 μm.) Full size image Heterozygous GBA1 mutations have been recognized as the strongest risk factor for PD and LB disorders [1] . In this study, we describe the generation and characterization of a collection of iPSC lines from GD patients, PD subjects harbouring heterozygous GBA1 mutations, as well as unaffected individuals. The cells used for iPSC generation in this study were obtained from donors harbouring L444P, RecNcil and N370S alleles. L444P and N370S point mutations are the most frequent GD-causing alleles that have been linked to PD [1] , [38] , whereas the RecNcil is a complex GBA-pseudogene recombinant allele composed of three point mutations, namely the 6433 T→C transition (L444P), 6468 G→C transition (A456P) and 6482 G→C transition (silent mutation). To identify PD phenotypes related to GBA1 mutations, isogenic gene-corrected iPSC lines were generated for each mutation. iPSCs were efficiently differentiated to mDA neurons without significant differences and enriched by FACS. For the first time, we report that iPSC neuronal differentiation recapitulates the developmental changes observed during human brain development and that enriched iPSC-derived neurons show the polysialoganglioside content of adult human brain. To examine the shift of the ganglioside pattern along in vitro differentiation of human iPSCs, we utilized a radioactive labelling method and compared the ganglioside composition of fibroblasts, iPSCs and iPSC-derived neurons before and after FACS enrichment. Unsorted iPSC-derived neurons showed an increased complexity of the ganglioside pattern compared with fibroblasts and iPSCs; however, they still had a high content of GM3, which is usually found at high levels in other cell types. Interestingly, unsorted neurons showed high levels of GD3, which is mainly associated with proliferating neural stem cells [16] . By contrast, despite the presence of low quantities of GM3 and GM2, the gangliosidic pattern of purified neurons mirrored the composition of human brain with GM1, GD1a, GD1b, GT1b as major compounds and GD3, GD2 and GQ1b in less abundance [39] . These findings show that using unsorted differentiated iPSCs, which are heterogeneous cell populations, significantly limits the analysis of disease-related pathways. This underlines the importance of cell sorting to reduce background noise in such experimental approaches [12] , [40] . Taken together, these data indicate that enriched iPSC-derived neurons represent a valuable tool to study the role of GSLs in neurodegeneration as well as in sphingolipidoses and disorders of brain development. In this context, we also show that the glycosyltransferases involved in the catabolic pathways of GSLs (GCase, GBA2, β-galactosidase, β-hexosaminidase) are upregulated on human iPSC neuronal differentiation. Activity and protein levels of these enzymes were almost absent in undifferentiated iPSCs, whereas mature neurons expressed high levels of such enzymes. This may suggest a key role of these glycohydrolases in brain development and maintenance of GSL pattern and composition in the adult human brain. GD patients with parkinsonism and PD patients carrying GBA1 mutations show classic PD pathology with widespread α-syn inclusions [41] . The exact mechanism is unknown, but GBA1 mutants may contribute to the enhanced aggregation of α-syn via a direct interaction [5] . In support of such a gain of function hypothesis, post-mortem studies in PD and LB disease, along with GD or GBA1 mutation carriers, have shown the presence of GCase in LBs and Lewy neurites [42] . Recent data suggest that loss of GCase activity may also lead to α-syn accumulation as a secondary effect of lysosomal dysfunction [25] , [27] and that the accumulation of Glc-Cer due to GCase deficiency induces increased α-syn oligomerization, which in turn decreases GCase activity [25] , [43] . By utilizing iPSC-derived neurons carrying heterozygous GBA1 mutations and their isogenic gene-corrected controls, we show that GBA1 mutations are directly linked to the increase of α-syn levels. For the first time, we report an increase of Glc-Cer in iPSC-derived neurons from PD patients carrying heterozygous GBA1 mutations, which may in turn influence α-syn levels and aggregation. Our data show that GBA1 mutations are linked to defects in the autophagic/lysosomal system characterized by an impairment of the autophagic flux with consequences for autophagosome clearance. Although we have observed an accumulation of lysosomes, the fusion between autophagosomes and lysosomes and the lysosomal hydrolytic function were impaired. This may explain the increased levels of α-syn in GBA1 mutant neurons and α-syn pathology in GBA-PD patients. Interestingly, the reduction in the glycohydrolase lysosomal activity in iPSC-derived neurons was accompanied by a reduction in the enzymatic activity of these enzymes in the CSFs of GBA-PD patients compared with control individuals. PD and parkinsonism have been described in many lysosomal storage diseases, suggesting that impairment of the endolysosomal compartment is strictly correlated with the onset of neuronal degeneration [44] . In this context, GBA1 mutations may alter the lysosomal function via several pathways. The intracellular lipid content strongly influences autolysosome formation as well as α-syn aggregation [15] , [45] . In contrast, increased levels of α-syn may cause lysosomal dysfunction in GBA1 mutant neurons via a positive feedback loop [25] . Furthermore, our data in isogenic controls, along with previous reports [46] , suggest the existence of a crosstalk between different enzymes involved in sphingolipid metabolism. Interestingly, we found that GBA2 enzyme activity was significantly decreased in iPSC-derived neurons harbouring GBA1 mutations. GBA2 is a non-lysosomal enzyme with glucosylceramidase function localized at the ER and plasma membrane [47] . It is encoded by the GBA2 gene and is highly expressed in the brain, testis and liver [48] . Notably, GBA2 mutations cause a form of autosomal-recessive cerebellar ataxia and have been recently linked to motor neuron defects in hereditary spastic paraplegia [49] , [50] . Mutant GCase in the ER leads to ER stress and induces the unfolded protein response in skin fibroblasts from GD patients and mutation carriers [51] . Since GBA2 is also located in the ER, such perturbations may affect its activity. Even though the mechanisms responsible for the observed impairment of GBA2 function remain unclear, our data show that the decrease in GBA2 enzymatic activity was reverted on ZFN-mediated GBA1 gene correction, suggesting a crosstalk between GCase and GBA2 activity. In favour of this hypothesis, a recent report shows that GBA2 activity depends on GCase, whereas GCase activity is independent of GBA2 (ref. 52 ). Further studies are needed to better elucidate such crosstalk and its role in disease onset and progression. GBA-PD and GD parental fibroblast lines showed an upregulation of the enzymatic activity of GBA2 and β-galactosidase compared with control cells. Such discrepancy can be attributed to the different sphingolipid metabolism in fibroblasts and neurons. As described above, neurons have high glycohydrolase enzymatic activity and a unique GSL content and distribution. Alternatively, even though only low passage fibroblasts were used in this study, such findings may also be due to the changes of the GSL pattern observed during subculture progression [21] . These data further support the importance of using iPSC-derived neurons as the ideal tool to model neurological diseases and in particular neurodegeneration associated with sphingolipidoses. In this study, we have generated a proteome profile of differentiated iPSCs. This is the first report of multiplexed quantitative proteomics being performed on a highly enriched neuronal fraction. As little as 15 μg for each cell line was used for quantitative proteomics using TMT labelling, leading to the identification of over 7,000 proteins from 12 LC-mass spectrometry runs. Such analysis enabled the identification of a protein, namely NECAB2, whose levels were increased in human iPSC-derived neurons harbouring mutations in the GBA1 gene. NECAB2 belongs to the family of neuronal calcium-binding proteins containing an N-terminal EF-hand domain (NECAB). It is highly expressed in the striatopallidal structures where it interacts with the adenosine A2A receptor [53] , [54] . Interestingly, a recently published microarray data set for putative novel mDA neuron-related transcription factors and membrane-associated proteins has shown that NECAB1 is a marker for mDA neurons, and it is highly expressed in the dorsal ventral tegmental area and dorsal substantia nigra [55] . Adult mDA neurons are autonomous pacemakers and rely on the activation of L-type Ca(V)1.3 calcium channels, leading to elevated intracellular calcium concentrations [56] . In addition, mDA neurons lack significant intrinsic calcium-buffering properties, which may explain their selective vulnerability to neurodegeneration [57] . A recent study demonstrates that the levels of calcium-binding proteins are reduced in cell bodies of neurons in areas selectively vulnerable to degeneration in PD. However, the surviving cells upregulate such proteins suggesting a compensatory mechanism [58] . Interestingly, we found increased basal levels of calcium and an increased calcium release from the ER on caffeine stimulation in GBA-PD and GD neurons. Such findings are in line with previous observations in pharmacological models of neuronopathic GD showing that Glc-Cer accumulation leads to overactivation of the ryanodine receptor [59] . The dysregulation of calcium homeostasis in diseased neurons was accompanied by an increased vulnerability to ER stress responses involving elevation of cytosolic calcium by the calcium ionophore A23187 and rotenone. Recently, mitochondrial impairment has been linked to GCase dysfunction providing a further rationale for the increased susceptibility to rotenone described in this study [60] . Importantly, increased neurotoxicity was observed in GBA1 mutant neurons exposed to A23187 on NECAB2 knockdown. These data demonstrate the calcium-buffering properties of NECAB2 and support the hypothesis that the increase of NECAB2 in neurons harbouring GBA1 mutations represents a compensatory mechanism in such vulnerable neurons. In summary our studies showed that both GD and PD iPSC-derived neurons have increased levels of α-syn and Glc-Cer as well as complex changes in the autophagic/lysosomal system and calcium homeostasis, which may underlie the selective vulnerability of mDA neurons to degeneration in PD. Taken together, our results suggest possible targets for the development of disease-modifying drugs for patients with familial and idiopathic PD. Sample collection Informed consent was obtained from all patients involved in our study before cell donation or CSF collection. The Ethics Committee of the Medical Faculty and the University Hospital Tübingen previously approved this consent form. PD was diagnosed according to UK Brain Bank criteria [61] . The open-reading frame (11 exons) of the GBA1 gene was entirely sequenced in cases and controls. See Supplementary Table 3 for primer sequences. For CSF studies, control individuals underwent spinal taps for exclusion of vascular events or inflammatory conditions. Any clinical sign of a neurodegenerative disorder led to exclusion from the study. Dermal fibroblasts were cultured in fibroblast medium, which consisted of DMEM (Biochrom) supplemented with 10% fetal calf serum, 1% penicillin/streptomycin/glutamine, 1% nonessential amino acids, 1% sodium pyruvate (all PAA) and 0.5 mM β-mercaptoethanol (Invitrogen). GD fibroblasts were obtained from the Telethon Genetic Biobank Network (02FFF0491979, 02FFF0352006, 02FFF0201995, 02FFF0361999). Generation of iPSCs and gene correction Fibroblasts were infected with a mix of retroviruses encoding OCT4, SOX2, KLF4 and c-MYC. Five days after infection, cells were split into six-well plates pre-seeded with irradiated mouse embryonic fibroblasts (MEF, GlobalStem). Seven days after infection the medium was changed to human embryonic stem cell (hESC) medium consisting of KO-DMEM (Gibco) supplemented with 20% KO-Serum Replacement (Invitrogen), 2 mM Glutamax (Invitrogen), 50 μM β-mercaptoethanol (Invitrogen), non-essential amino acids (Cambrex) and 10 ng ml −1 b-FGF (Peprotech). Individual colonies were isolated and clonally expanded on MEFs. For gene correction, iPSCs were dissociated into single cells using Accutase (PAA). In total, 1.5 × 10 6 cells were diluted in hESC medium and collected by centrifugation. Cells were transfected with 0.83 μg of each ZFN construct (Sigma), as well as 3.3 μg linearized targeting vector, using the Stem cell Nucleofection Kit and the Amaxa Nucleofector I (both Lonza), according to the manufacturer’s instructions (program B16). The transfected cells were replated onto MEF-coated plates in hESC medium supplemented with 10μM ROCK inhibitor Y27632 (Ascent Scientific). From day 2 on, medium was changed on a daily basis. After colony formation (5–7 days), 250 μg ml −1 G418 (Biochrom) was added to select for homologous recombined clones. Resistant colonies were transferred to 12-well plates and expanded on MEFs for further characterization. To confirm gene correction, genomic DNA was extracted from the gene-targeted clones and sequenced at the corresponding locus. Final characterization was achieved by extraction of RNA using the RNeasy kit (Qiagen), transcription into cDNA and sequencing of the cDNA. See Supplementary Table 4 for primer sequences. Karyotyping Karyotyping was performed by G-banding to examine the integrity of the chromosomes by the Cytogenetics Laboratory at the University of Tübingen. In vitro differentiation of human iPSCs To test in vitro pluripotency, embryoid bodies (EBs) were generated from iPSCs by culturing the colonies in hESC medium in the absence of b-FGF. After 5 days, EBs were transferred to gelatin-coated plates and subsequently cultured for another 14 days in N2/B27 supplemented with 10 μM SB431542 (Tocris) (ectoderm) or knockout DMEM (Invitrogen) supplemented with 20% FBS, 1 mM L -glutamine ( L -glut), 1% non-essential amino acids, 0.1 mM β-mercaptoethanol and 1% penicillin/streptomycin (endoderm/mesoderm). After 2 weeks, cultures were fixed and stained as indicated. Teratoma assay Teratoma assays were performed by Applied Stem Cell (Menlo Park) [62] . In brief, 10 6 iPSCs were injected into the kidney capsule and testis of Fox Chase SCID-beige mice. Animals were killed ~\n6–12 weeks after injection and haematoxylin-eosin (H&E) stainings were used to analyse harvested tissues. Differentiation of iPSCs into midbrain DA neurons iPSCs were differentiated into DA neurons following a floor plate-based mDA neuron induction protocol [10] , with minor modifications. iPSC colonies were dissociated into a single-cell suspension using Accutase and 10 μM ROCK inhibitor Y-27632. Cells were collected by centrifugation and seeded at a density of 1.5 × 10 5 cells per well on Matrigel (BD Biosciences)-coated 12-well plates. Differentiation was based on exposure to LDN193189 (100 nM, Stemgent) from days 0–11, SB431542 (10 μM, Tocris) from days 0–5, SHH C25II (100 ng ml −1 , R&D), purmorphamine (2 μM, EMD) and FGF8 (100 ng ml −1 , Peprotech) from days 1–7 and CHIR99021 (CHIR; 3 μM, Stemgent) from days 3–13. Cells were grown for 11 days on Matrigel in knockout serum replacement medium (KSR) containing KO-DMEM, 15% knockout serum replacement, 2 mM L -glutamine and 10 μM β-mercaptoethanol. KSR medium was gradually shifted to N2 medium starting on day 5 of differentiation. On day 11, media was changed to Neurobasal/B27/ L -glut containing medium (NB/B27; Invitrogen) supplemented with CHIR (until day 13), BDNF (brain-derived neurotrophic factor, 20 ng ml −1 ; R&D), ascorbic acid (0.2 mM, Sigma), GDNF (glial cell line-derived neurotrophic factor, 20 ng ml −1 ; R&D), TGFβ3 (transforming growth factor type β3, 1 ng ml −1 ; R&D), dibutyryl cAMP (dbcAMP, 0.5 mM; Sigma) and DAPT (10 μM; Tocris,) for 9 days. On day 21, cells were dissociated using Accutase and replated on dishes pre-coated with poly- L -ornithine (PLO; 15 μg ml −1 ) and laminin (1 μg ml −1 ) in differentiation medium (NB/B27+BDNF, ascorbic acid, GDNF, dbcAMP, TGFβ3 and DAPT). Quantitative Real-Time PCR Total RNA was extracted with an RNeasy kit and quantitative RT–PCR reaction was performed using the SYBR GREEN Kit (Qiagen). The expression level of each gene was normalized to endogenous HMBS levels. Fold-change in gene expression was calculated using the 2 −ΔΔCT method, based on biological reference samples and housekeeping genes for normalization. All the results were obtained from the evaluation of three technical replicates of three independent experiments. See Supplementary Table 5 for primer sequences. Flow cytometry Cells were harvested and gently dissociated using TrypLE (Life Technologies) to obtain a single-cell suspension of 0.5–2 × 10 6 cells ml −1 and resuspended in Ca 2+ /Mg 2+ free phosphate buffered saline (PBS; PAA Laboratories) with 2% FBS and distributed into 1.5 ml microcentrifuge tubes. Centrifugation steps were conducted using a refrigerated table microcentrifuge (Peqlab Perfect Spin 24 R) at 2,400 r.p.m. (542 g) for 3–5 min. Surface antigens were labelled by incubating with the primary antibodies for 30 min in the dark at room temperature. The following conjugated primary antibodies were used in the study: CD15-FITC, CD29-FITC, CD44-FITC, CD24-PE, CD184-APC. See Supplementary Table 6 for the list of antibodies. All antibodies were carefully titrated. The stained cells were analysed on a BD Accuri C6 benchtop cytometer equipped with FL1 (533/30), FL2 (585/40) and FL4 (675/25) bandpass filters. Data were analysed and are presented using BD CFlow software version 1.0.227.4. Neuronal cell sorting was performed on a Beckman Coulter MoFlo instrument using a 100 μm nozzle and sheath pressure of 20 to 25 psi (ref. 11 ). Excluding debris and the minor amount of cells observed to be dead after harvesting, a primary gate based on forward and side scatter was set to select the overall population of interest. FSC-peak (height) versus FSC-integral (area) gating was applied to exclude doublets for cell sorting. Gates for detecting positive staining were set against unstained controls for surface antigens. Where appropriate, compensation was applied according to single-stained controls of the same cell type included in each individual experiment. Electrophysiology For whole-cell patch clamp experiments, neurons derived from iPSCs were plated on 35 mm petri-dishes (Greiner-bio-one). Recordings of cultured neurons were performed at room temperature using an Axopatch 200B amplifier (Molecular devices). Data were digitized using a DigiData 1320A (Molecular devices). During electrophysiological recordings, cells were kept in extracellular solution containing (in mM): 142 NaCl, 8.09 KCl, 6 MgCl 2 , 1 CaCl 2 , 10 glucose, 10 HEPES and a final pH of 7.4. Patch pipettes were pulled from borosilicate glass (Science products) using a Sutter P97 Puller (Sutter Instruments Company). Their resistance ranged from 3 to 5 MΩ. Patch pipettes were filled with intracellular solution containing (in mM): 5 KCl, 4 ATP-Mg, 10 phosphocreatine, 0.3 GTP-Na, 10 HEPES, 125 K-gluconate, 2 MgCl 2 , 10 EGTA with a final pH of 7.2 and an osmolarity of 290 mosmol. The sampling rate was 50 kHz and data were low-pass filtered at 10 kHz. Series resistance (<20 MΩ) was monitored during the experiment. Cells showing unstable series resistance or resting membrane potential were discarded. HPLC analysis Differentiated neuronal cultures at DIV65 of differentiation were washed once with HBSS and then treated with 56 mM KCl in HBSS for 30 min; control cultures were exposed to HBSS. Supernatants were collected, snap-frozen and stored at −80 °C until analysis. Concentrations of DA were determined by column liquid chromatography with electrochemical detection. The HPLC system (HTEC-500, Eicom Corp.) including a pulse-free microflow pump, a degasser and an amperometric detector equipped with a glassy-carbon electrode, operating at +0.45 V versus an Ag/AgCl electrode, was used. Samples were injected by use of a CMA/200 Refrigerated Microsampler (CMA/Microdialysis). The chromatograms were recorded and integrated by a computerized data acquisition system (DataApex). DA was separated on a 150 × 2.1 i.d. mm column (CA5-ODS, Eicom Corp.). The mobile phase consisted of 0.1 M phosphate buffer at pH 6.0, 0.13 mM EDTA, 2.3 mM sodium-1-octanesulfonate and 20% methanol. The detection limit (signal-to-noise ratio=3) for DA was estimated to 0.5 fmol in 15 μl (0.03 nM) injected onto the column. Well to well variations were adjusted by concentration of cleared protein lysates. Glc-Cer and Gal-Cer analysis by mass spectrometry Quantitative analysis of Glc-Cer was carried out by LC-MS/MS. In brief, frozen cell pellets were suspended in 50 μl of water and extracted with 1 ml of a solution of acetonitrile: methanol: water (97:2:1, v v −1 v −1 ) at room temperature. Extracts were injected onto an Atlantis HILIC silica column (Waters Corp.) for separation of Glc-Cer and Gal-Cer, and respective molecules were detected using MRM mode tandem mass spectrometry with an AB Sciex API-5000 mass spectrometer. Analytes were quantitated against standard curves using standards obtained from Matreya, LLC (Pleasant Gap). Enzymatic activity assays Total cell associated GCase activities were analysed using 4-methylumbelliferyl-β- D -glucopyranoside (MUB-Glc), β-galactosidase and β-hexosaminidase activities were assayed using the artificial substrates 4-methylumbelliferyl β- D -galactopyranoside (MUB-Gal) and 4-methylumbelliferyl N-acetyl-β- D -glucosaminide (MUG) (all Glycosynth) [30] . Differentiated iPSCs at DIV65-70 were enriched by FACS and plated into Matrigel-coated 48-well assay plates in differentiation medium (500 μl per well). Media was changed every 3 days. Seven days after plating, cells were washed twice with PBS, harvested and lysed in water containing complete protease inhibitor cocktails (Roche). Total cell protein was measured using the Micro BCA assay reagent (Pierce). Cell lysates were transferred to a 96-well microplate and enzymatic assays were performed in triplicates. The activities of β-galactosidase and β-hexosaminidase were measured in McIlvaine Buffer (0.1 M Citrate/0.2 M Phosphate) pH 5.2 using 0.5 mM MUB-Gal and 1 mM MUG, respectively. For CBE-sensitive GCase and GBA2 assays, the cells were pre-incubated for 30 min at room temperature in McIlvaine Buffer (0.1 M Citrate/0.2 M Phosphate) pH 6.0 containing 5 nM AMP-DNM N -(5-adamantane-1-yl-methoxy-pentyl)-deoxynojirimycin) [24] and 1 mM CBE (conduritol B epoxide, Calbiochem), respectively. GCase and GBA2 activities were also determined using 150 nM AMP-DNJ (Miglustat, Zavesca) as an inhibitor (no significant differences were found compared with AMP-DNM). No enzymatic activity was detected after the concomitant use of CBE and AMP-DNM or AMP-DNJ. After incubation with the inhibitors, MUB-Glc was added at a final concentration of 3 mM. The reaction mixtures were incubated at 37 °C under gentle shaking. The fluorescence was recorded after transferring 20 μl of the reaction mixtures to a microplate and adding 180 μl of 0.25 M glycine, pH 10.7. Data were calculated as pmoles of converted substrate mg −1 of cell protein h −1 . Sphingolipid analyses Fibroblasts, undifferentiated iPSCs, differentiated iPSCs, sorted neurons and granule cells obtained from the cerebellum of 8-day-old Harlan Sprague–Dawley rats at DIV 8 were plated on poly- L -ornithine (PLO)/laminin-coated 48 wells. Two days (fibroblasts, undifferentiated iPSCs and primary granule cells, unsorted differentiated iPSCs) or seven days (sorted neurons) after plating, cells were incubated with 3 × 10 −8 [1- 3 H]- D -erythro-C18/C20-sphingosine in the appropriate culture medium (2-h pulse followed by a 48-h chase). Fresh brains from three 2-month-old C57BL/6j mice and three Harlan Sprague–Dawley rats were weighted, minced with a razor blade, homogenized in iced water (500 mg of fresh tissue ml −1 ), sonicated and then lyophilized. Lipids were extracted from cells and brains with chloroform/methanol/water in the ratio 2:1:0.1 by volume and subjected to a two-phase partitioning. Radioactive gangliosides were separated by mono- or two-dimensional HPTLC carried out with the solvent systems chloroform/methanol/0.2% aqueous CaCl 2 , 50: 42: 11 or 55: 45: 10 [63] . Brain endogenous gangliosides were recognized using Ehrlich’s reagent [64] . Radioactive lipids were identified and quantified with a Beta-Imager 2000 instrument (Biospace) using an acquisition time of about 48 h. The use of animal models was approved by the Italian Government (D.M. 33/2004). Immunofluorescence Cells were fixed in 4% paraformaldehyde for 10 min, rinsed with PBS and blocked by 10% normal goat or donkey serum in PBST (PBS+0.1% TritonX-100) for 60 min [62] . Alkaline phosphatase staining was performed using the Alkaline Phosphatase Kit (Millipore), according to the manufacturer’s protocol. For LC3, LAMP1 and LAMP2 analysis, cells were co-stained for β-TubIII and TH, and images were acquired with a Zeiss LSM 510 (Carl Zeiss) confocal microscope using a 63 × 1.4NA plan-apochromat oil objective. Images were processed in ImageJ (NIH) and brightness/contrast was adjusted equally. The particle size and number in β-TubIII and TH + cells were quantified with the ‘analyse particles’ plug-in in ImageJ (NIH). Quantification was carried out on at least 50 cells per condition from independent experiments. Co-localization of LC3/LAMP1 in TH + neurons was quantified in threshold images with the ‘JACoP’ plug-in of the ImageJ software. See Supplementary Table 6 for the list of antibodies used. Protein extraction and western blotting Proteins were extracted using RIPA protein extraction buffer (50 mM Tris pH 8, 150 mM NaCl, 0.5% natriumdeoxycholate, 1% NP40, 0.1% SDS) containing protease and phosphatase inhibitors (Roche) on ice. In total, 15–30 μg of the protein lysate was loaded on a 4–12% Bis-Tris Gel (NuPAGE, Invitrogen) and transferred on a PVDF membrane (Millipore). Blots were incubated with primary antibodies overnight at 4 °C on a shaker platform and were then probed with anti-mouse (Dianova), anti-rabbit (Dako) or anti-goat (JacksonLab) IgG-HRP (H+L) secondary antibody (all 1:10.000) for 1 h at room temperature. Visualization was done by using Amersham ECL Western Blotting Detection Reagent (GE Healthcare). Densitometry analyses on the immunoblots from multiple experiments were performed by ImageJ software. See Supplementary Table 6 for the list of antibodies used. Full-length images of immunoblots are shown in Supplementary Figs 16–18 . Autophagy studies Where indicated, cells were treated with NH 4 Cl (20 mM) and leupeptin (200 μM) (EMD, Millipore) for 4 h and then fixed or lysed for western blot analysis. LC3-II levels were quantified by densitometry and normalized for β-actin. LC3 flux was quantified by dividing levels of LC3-II after lysosomal inhibitor treatment for 4 h by the level of LC3-II without treatment. Calcium imaging Cells were loaded with Fura-2 acetoxymethyl ester (Sigma) for 30 min at RT in recording medium (NaCl 140 mM, KCl 4 mM, CaCl 2 2 mM, MgCl 2 1 mM, Glucose 4 mM, HEPES 10 mM). KCl (60 mM) and caffeine (10 mM, Sigma) were prepared in recording medium. For baseline recordings, scans were acquired every 10 s for 5 min. Fluorescence measurements were obtained on an epifluorescence inverted microscope (Zeiss Axio Observer). All imaging data were collected and analysed using AxioVision (rel. 4.8) software. Cytotoxicity assays After 63–65 days in vitro , cells were plated on PLO/laminin-coated 96-well plates at a density of 30.000 cells per well. Two days later, cells were incubated with A23187 (1 to 5 μM, Tocris), or rotenone (50 to 200 nM, Sigma) in N2 medium for 4 h and 24 h, respectively. Dimethyl sulfoxide (DMSO) was used as vehicle and control conditions. The LDH assay (Promega) was performed as per the manufacturer’s instructions. For knockdown experiments, cytotoxicity assays were performed 72 h after non-targeting shRNA or NECAB2 shRNA lentiviral infection. Proteomic analysis Cells were resuspended in 100 μl lysis buffer (8 M urea, 5 mM DTT, 50 mM HEPES pH 8.5, 1 × Roche Protease Inhibitors, 1 × Roche PhosphoStop phosphatase inhibitors) and cell debris was removed by centrifugation (10 min, 9,000 g ). The clarified lysate was allowed to incubate at room temperature for 30 min for reduction of disulphide bonds. Cysteines were then alkylated with 15 mM iodoacetamide (45 min, RT, dark). Excess iodoacetamide was quenched with DTT (15 min, RT, dark). The proteins were precipitated using methanol-chloroform and then resuspended in a small volume of 8 M urea, 50 mM HEPES pH 8.5. Before digestion, they were diluted to 1 M urea, 50 mM HEPES pH 8.5. The protein concentrations were measured using the BCA assay (Pierce). Samples were digested overnight at 37 °C with trypsin, which was added at a 1:100 protease-to-protein ratio. This reaction was subsequently quenched with 1% formic acid, the sample desalted using C18 solid-phase extraction (Sep-Pak, Waters) and then dried by vacuum-centrifugation. To perform tandem mass tag labelling, desalted peptides were resuspended in 35 μl of 100 mM HEPES pH 8.5 and 8 μl of acetonitrile. TMT reagents (0.8 mg) were dissolved in anhydrous acetonitrile (40 μl) of which 4 μl was added to the peptides. The mixture was incubated at room temperature for 1 h. The labelling reaction was then quenched by the addition of hydroxylamine to a final concentration of 0.3% (v/v). Each of the TMT-labelled samples were combined at a 1:1:1:1:1:1:1 ratio, dried, desalted and fractionated using high pH reversed-phase (HPRP). Following fractionating the samples were acidified to 1% formic acid (v/v), dried, desalted using StageTips, dried and then reconstituted in 5% acetonitrile and 5% formic acid. LC-MS/MS was performed on an LTQ Orbitrap Elite mass spectrometer (Thermo-Fisher Scientific) [65] . The total LC-MS run length for each sample was 180 min consisting of a 150 min gradient from 6 to 33% acetonitrile in 0.125% formic acid. A recently developed MS3 method was used to overcome the interference problem in acquisition of TMT data [66] . Data analysis Mass spectrometry data were processed using an in-house software pipeline [67] . Raw files were converted to mzXML files and searched using the Sequest algorithm [68] against a composite database containing all sequences from the human International Protein Index (IPI) database (version 3.6) in forward and reverse orientations. Database searching matched MS/MS spectra with fully tryptic peptides from this composite database with a precursor ion tolerance of 20 p.p.m. and a product ion tolerance of 1 Da. Carbamidomethylation of cysteine residues (+57.02146 Da) and TMT tags on peptide N-termini (+229.162932 Da) were set as static modifications. Oxidation of methionines (+15.99492 Da) was set as a variable modification. Linear discriminant analysis was used to filter peptide spectral matches to a 1% FDR, as described previously [67] . For analysis of TMT data, the reporter ion counts of the peptide spectral matches for each protein were summed, as described previously [66] , [69] . Statistical significance was calculated by t -test analysis adjusted using the Benjamini and Hochberg method to control for false-discovery rate and filtered for proteins whose levels changed by at least 1.2-fold. Expression changes were considered significantly up- or downregulated when the P -value was ≤0.05. Cerebrospinal fluid enzyme assays Total protein amounts were measured using a DC protein assay in triplicate according to the manufacturer’s instructions (Biorad). β-Glucosidase activities were analysed by using 4-methylumbelliferyl-β- D -glucopyranoside (MUB-Glc). β-Galactosidase and β-hexosaminidase activities were assayed by using the artificial substrates 4-Methylumbelliferyl β- D -galactopyranoside (MUB-Gal) and 4-Methylumbelliferyl N-acetyl-β- D -glucosaminide (MUG). β-Mannosidase, α-mannosidase and α-fucosidase activities were determined using 4-methylumbelliferyl-β- D -mannopyranoside (MUB-β-Man), 4-methylumbelliferyl-α- D -mannopyranoside (MUB-α-Man) and 4-methylumbelliferyl-α-L-fucopyranoside, respectively (MUB-Fuc) (all Glycosynth). Same amounts of CSF protein was transferred to a 96-well microplate and enzymatic assays performed in triplicate. Determination of the β-galactosidase, β-hexosaminidase, β-mannosidase, α-mannosidase and α-fucosidase activities were performed in McIlvaine Buffer (0.1 M Citrate/0.2 M Phosphate) pH 5.2 using 0.5 mM MUB-Gal and 3 mM MUG, 3 mM MUB-β-Man, 3 mM MUB-α-Man and 3 mM MUB- Fuc, respectively. For CBE-sensitive β-glucosidase and GBA2 assays, cells were pre-incubated for 30 min at room temperature in McIlvaine Buffer (0.1 M Citrate/0.2 M Phosphate) pH 6.0 with 5 nM AMP-DNM and 1 mM CBE, respectively. The activity of the CBE-sensitive β-glucosidase was determined in the presence of 0.5% Triton X-100. After 30 min, MUB-Glc was added at a final concentration of 6 mM. After 30 to 180 min of incubation at 450 r.p.m. stirring and 37 °C, fluorescence was detected by transferring 20 μl of the reaction mixtures to a microplate and adding 180 μl of 0.25 M glycine, pH 10.7. Lentivirus-mediated shRNA The verified Mission lentiviral plasmids encoding turbo GFP (SHC003), non-targeting shRNA (SHC016) and NECAB2 shRNA (TRCN0000056234, TRCN000056236) in pLKO.1-puro vector backbone were purchased from Sigma-Aldrich. Lentiviral stocks were prepared by calcium phosphate transfection and the packaging vectors pLP1, pLP2 and pLP/VSVG using the ViraPower HiPerform T-REx Gateway Expression System (Invitrogen). In brief, 80% confluent HEK 293T cells were transfected with 3 μg of plasmid DNA and 9 μg of the ViraPower packaging mix using the TransIT-LT1 Transfection Reagent (Mirus). The following day, the medium was replaced with fresh culture medium and cells were incubated at 37 °C in a humified 5% CO 2 incubator. After 48 h, medium was changed and the virus-containing supernatant was harvested, filtered through a 0.45 μm PVDF filter membrane (Millipore) and concentrated by centrifugation in a Vivaspin column (Sartorius Stedim Biotech) at 4,000 r.p.m. at 4 °C for 15 min. Supernatants were collected over 48 to 60 h and titred used at an MOI of five to infect cells. Statistical analysis The Statistical Package GraphPad Prism version 4.00 (GraphPad Software, San Diego California USA) was used to analyse the data. Statistical testing involved a two-tailed paired or unpaired Student’s t -test, One-way Anova with Bonferroni’s multiple comparison test or Mann–Whitney U test, as appropriate. Data are expressed as mean+s.e.m. (or+s.d.) as indicated. Significance was considered for P <0.05. Accession codes The mass spectrometry proteomics data have been deposited in ProteomeXchange via the PRIDE partner repository [70] under the accession code PXD000866. How to cite this article: Schöndorf, D. C. et al. iPSC-derived neurons from GBA1-associated Parkinson’s disease patients show autophagic defects and impaired calcium homeostasis. Nat. Commun. 5:4028 doi: 10.1038/ncomms5028 (2014).